A systematic analysis of the PARP protein family identifies new functions critical for cell physiology The poly(ADP-ribose) polymerase (PARP) family of proteins use NAD + as their substrate to modify acceptor proteins with ADP-ribose modifications. The function of most PARPs under physiological conditions is unknown. Here, to better understand this protein family, we systematically analyse the cell cycle localization of each PARP and of poly(ADP-ribose), a product of PARP activity, then identify the knockdown phenotype of each protein and perform secondary assays to elucidate function. We show that most PARPs are cytoplasmic, identify cell cycle differences in the ratio of nuclear to cytoplasmic poly(ADP-ribose) and identify four phenotypic classes of PARP function. These include the regulation of membrane structures, cell viability, cell division and the actin cytoskeleton. Further analysis of PARP14 shows that it is a component of focal adhesion complexes required for proper cell motility and focal adhesion function. In total, we show that PARP proteins are critical regulators of eukaryotic physiology. Post-translational protein modifications such as phosphorylation, ubiquitination and acetylation are critical for regulating acceptor protein function [1] . A less well-understood modification is ADP-ribosylation, in which units of ADP-ribose (ADPr) are added onto acceptor proteins using NAD + as substrate [2] . Proteins can be modified by polymers of ADPr (poly(ADP-ribose) (PAR)), which vary in length and extent of branching, or by shorter modifications such as mono(ADP-ribose) (MAR). The best known functions of ADP-ribosylation occur during regulation of cell stress responses such as DNA damage [3] , apoptosis [4] , heat shock [5] , cytoplasmic stress [6] and the unfolded protein response [7] . However, it has become increasingly clear that ADPr modifications are critical for cell physiology under non-stress conditions, because cell division [8] , [9] , [10] , [11] , transcription and chromatin structure regulation [12] , [13] all require ADP-ribosylation. PAR polymerases (PARPs; also known as ADP-ribosyl transferases (ARTDs)) are a family of enzymes found in eukaryotes and prokaryotes that generate ADPr modifications onto acceptor proteins [2] , [12] , [14] . 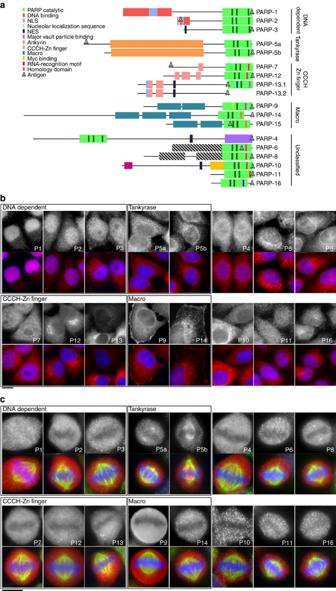Figure 1: PARPs localize throughout the cell. (a) Domain structure of PARP proteins. Functional domains are indicated, and green dashes within the catalytic domain indicate H-Y-E amino acids thought to be required for PAR synthesis activity. Dashes with different colours indicate the replacement of these amino acids with the following residues: I (red), Y (blue), V (purple), Q (yellow), T (pink) and L (orange). (b,c) HeLa cells were fixed and then stained with affinity-purified antibodies generated against each PARP. Data are presented in PARP subfamily groupings and labelled in boxes, with each PARP labelled as P(x). A summary of localization patterns is provided inTable 1. (b) Interphase localization of PARP proteins. Most PARPs are cytoplasmic (top). Merge (below) shows PARP (red) and Hoechst 33342 staining (blue). (c) PARP localization in mitotic cells (top). A subset of PARPs localize to the mitotic spindle (P5a, 5b, 8 and 11). Merge (below) shows PARP (red), tubulin (green) and Hoechst 33342 (blue) staining. Scale bars, 10 μm. See alsoSupplementary Figs S1–S3andTables 1,2. Humans are thought to express 17 PARPs identified on the basis of sequence homology to the catalytic domain of PARP1 (refs 15 , 16 ) (for a summary of PARP/ARTD nomenclature, see Table 1 ). The PARP family is further grouped into four subfamilies based on the presence of functionally characterized domains in regions outside the PARP domain: DNA-dependent PARPs , initially thought to require DNA binding for enzymatic activity; tankyrases , with protein-binding ankyrin repeats; CCCH zinc finger PARPs that contain CCCH zinc finger domains shown to bind viral RNA; and macro PARPs , with ADPr-binding macro domains [17] . The remaining PARPs are referred to as unclassified PARPs . A diagram of the PARPs, including motifs and domains, is provided in Fig. 1a (a more thorough description of the PARP family is reviewed in refs 11 , 12 , 18 , 19 ). Both the expression pattern of the various PARPs in human somatic cells and the physiological function of the majority of PARPs have not been established. Table 1 Summary of PARP family localization and knockdown phenotypes. Full size table Figure 1: PARPs localize throughout the cell. ( a ) Domain structure of PARP proteins. Functional domains are indicated, and green dashes within the catalytic domain indicate H-Y-E amino acids thought to be required for PAR synthesis activity. Dashes with different colours indicate the replacement of these amino acids with the following residues: I (red), Y (blue), V (purple), Q (yellow), T (pink) and L (orange). ( b , c ) HeLa cells were fixed and then stained with affinity-purified antibodies generated against each PARP. Data are presented in PARP subfamily groupings and labelled in boxes, with each PARP labelled as P(x). A summary of localization patterns is provided in Table 1 . ( b ) Interphase localization of PARP proteins. Most PARPs are cytoplasmic (top). Merge (below) shows PARP (red) and Hoechst 33342 staining (blue). ( c ) PARP localization in mitotic cells (top). A subset of PARPs localize to the mitotic spindle (P5a, 5b, 8 and 11). Merge (below) shows PARP (red), tubulin (green) and Hoechst 33342 (blue) staining. Scale bars, 10 μm. See also Supplementary Figs S1–S3 and Tables 1 , 2 . Full size image Based on the experimental study of a subset of PARPs combined with bioinformatic analysis, each PARP is predicted to exhibit either MAR or PAR synthesis activity or catalytic inactivity [20] . Sequence analysis predicts that DNA-dependent PARPs, tankyrases and PARP4 generate PAR, PARP9 and 13 are catalytically inactive, and all other PARPs generate MAR [20] . Specific amino acid residues that have been identified as targets of PARP modification include glutamic acid, aspartic acid and lysine residues [21] . To better understand the PARPs and PAR, we performed a system-level analysis of each PARP protein and the PAR polymer, examining localization and expression throughout the cell cycle. We then examined the knockdown phenotype of each PARP and performed follow-up analyses to help elucidate function. This work identifies new physiological functions for the PARP family, including the regulation of cell viability, cellular membrane structures and the actin cytoskeleton. Finally, we closely examined the function of PARP14, a member of the actin cytoskeleton-regulating macro PARPs. We report that PARP14 is a component of focal adhesion (FA) complexes that regulates the strength and stability of cellular attachment to substrate. Most human PARPs are expressed and most are cytoplasmic To examine PARP expression levels in human somatic cells, we analysed transcript abundance using Illumina RNA sequencing of HeLa cells originally derived from transformed cervical cancer cells, and retinal primary epithelial (RPE1) cells immortalized via human telomerase reverse transcriptase (hTERT) expression. 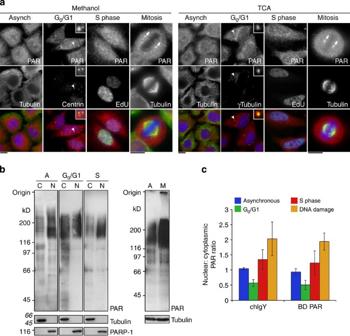Figure 2: Poly(ADP-ribose) is localized to the cytoplasm and nucleus throughout the cell cycle. (a) Asynchronous populations of HeLa cells (Asynch) or cells arrested in G0/G1, S phase or mitosis were fixed with MeOH or TCA and then stained for PAR (Tulip chIgY), and Centrin or γ-Tubulin, to identify single centriole pairs found during Go/G1, EdU, incorporated during S phase, and Tubulin, to stain mitotic spindles. In asynchronous cells and during Go/G1, S phase and mitosis, PAR staining was punctate with strong staining at the centrosome (arrowhead) and poles of the mitotic spindle (arrows). S-phase cells exhibited increased punctate staining in the nucleus relative to Go/G1cells. Merge shows PAR (red), cell cycle markers (green) and Hoechst 33342 (blue). Scale bars, 10 μm. (b) Cytoplasmic (C) and nuclear (N) extracts prepared from identical cell pellets, then normalized to cell volume, were generated from asynchronous, Go/G1and S-phase-arrested cells. Extracts were immunoblotted with Tulip chIgY anti-PAR antibody. Cytoplasmic and nuclear extracts were further examined for the presence of tubulin, a cytoplasmic protein, or PARP1, a nuclear protein, to assay for contamination between the fractions. Total cell extracts were also prepared from asynchronous (A) and mitotic (M) cells and immunoblotted with Tulip chIgY anti-PAR antibody. Positions of molecular-weight markers are indicated on the right in black, and molecular weights shown in italics identify the closest markers above and below the cropped region. (c) Quantitation of signal intensity of PAR immunoblots using chIgY and BD PAR antibodies. The ratio of nuclear to cytoplasmic PAR increases during S phase and DNA damage. The integrated intensity over the entire lane was determined, and the ratio of nuclear:cytoplasmic signal was calculated. Error bars represent s.d.,n=3. See alsoSupplementary Fig. S5. Fragments per kilobase of transcript per million fragments mapped values for each PARP, PAR glycohydrolase (PARG), a PAR hydrolysing enzyme and standard normalizing controls (actin and glyceraldehyde 3-phosphate dehydrogenase), are shown in Table 2 . With the exception of PARP15 (omitted from subsequent analyses), all PARPs were expressed in both epithelial cell lines, with relative expression levels varying by several orders of magnitude. Table 2 PARP transcript levels. Full size table Localization was then analysed using a library of N-terminal green fluorescent protein (GFP) fusions and affinity-purified peptide antibodies generated for each PARP. Specificity of each reagent was cross-verified by staining and blotting GFP-PARP-expressing HeLa cells with corresponding anti-PARP antibodies ( Supplementary Fig. S1 ). GFP-PARP-expressing cells exhibited overlapping GFP and antibody staining patterns when fixed and stained with anti-PARP antibody ( Supplementary Fig. S1A,B ). To further confirm that the N-terminal GFP fusions did not disrupt PARP localization, we analysed the localization of N-terminal fusions of the much smaller streptavidin-binding peptide (38 amino acid) to select PARPs. SBP-PARP and GFP-PARP localization patterns were identical ( Supplementary Fig. S1C ). In general, expression of GFP-PARP fusions did not result in cellular phenotypes, however, instances where phenotypes were detected are noted below. PARP antibodies verified in this manner were then used to stain interphase ( Fig. 1b ) and mitotic ( Fig. 1c ) cells. Localization was highly similar in HeLa and hTERT-RPE1 cells ( Fig. 1 , Supplementary Fig. S2 ). Cell cycle localization was then analysed in RPE1 cells arrested in G o /G 1 , S phase and mitosis ( Supplementary Fig. S2B–D ). Cell cycle state was confirmed via centrin staining, to identify single centriole pairs present in G o /G 1 (ref. 22 ), EdU labelling for S phase and tubulin staining to identify mitotic spindles present during mitosis. Most PARPs were cytoplasmic throughout the cell cycle, exhibiting additional enrichment at specific organelles. Six PARPs from three subfamilies localized to the centrosome: PARP2 and 3 in G o /G 1 ( Supplementary Fig. S2B ; centrosomal localization for PARP3 and 5a was previously identified [23] , [24] ); PARP11 and PARP5b during mitosis ( Supplementary Fig. S3A ); and PARP5a and 8 throughout the cell cycle ( Supplementary Fig. S3A ). Multiple PARPs and the previous identification of PARG at this site [25] suggest that ADPr is actively regulated there. Five PARPs from three subfamilies localized to membranous organelles: PARP8 to nuclear envelope, PARP12 to Golgi ( Supplementary Fig. S3B ), PARP9 and 14 to plasma membrane ( Supplementary Fig. S3C ) and PARP16 to endoplasmic reticulum ( Supplementary Fig. S3D ). Finally, four PARPs from two subfamilies localized to the mitotic spindle: PARP5a and 5b and unclassified PARP8 and 11 localized to spindle poles [9] , [10] , [24] ( Supplementary Fig. S3A ). PARP localization, largely consistent with knockdown phenotypes, is summarized below and in Table 1 . All DNA-dependent PARPs were nuclear during interphase, with PARP2 and 3 exhibiting additional cytoplasmic localization ( Fig. 1b ). Consistent with previous studies [23] , [26] , PARP3 localization varied with the cell cycle, with centrosomal and nuclear enrichment in G o /G 1 and cytoplasmic enrichment in S phase ( Supplementary Fig. S2B,C ). During mitosis, PARP1 was enriched at chromatin, and PARP2 and 3 were cytoplasmic ( Fig. 1c , Supplementary Fig. S2D ). Both tankyrases localized to cytoplasmic puncta during interphase ( Fig. 1b ). During mitosis, PARP5a and 5b localized to the mitotic spindle pole [9] , [27] . We identified additional localization for PARP5b throughout the spindle ( Fig. 1c , Supplementary Fig. S2D ). The CCCH Zn-finger PARPs were primarily cytoplasmic during interphase, exhibiting punctate localizations ( Fig. 1b ). In addition, PARP7 localized to nuclear foci, PARP12 exhibited juxtanuclear localization resembling Golgi staining and PARP13 exhibited a ∼ 4–5-fold variability in expression between clusters of cells, suggesting clonal variability ( Fig. 1b ). Cells expressing high concentrations of GFP-PARP12 and 13 assembled stress granules in the cytoplasm as previously described [6] . PARP12 localization to the Golgi was confirmed by co-localization with trans Golgi protein p230 ( Supplementary Fig. S3B ). Overexpression of GFP-PARP12 blocked PARP12 localization to the Golgi and disrupted Golgi structure, analysed via staining of p230, a trans Golgi marker ( Supplementary Fig. S4A,B ). Although p230 staining intensity was unaltered in cells overexpressing GFP-PARP12, Golgi area increased ∼ 1.58-fold relative to control cells. No such defects were found in untransfected, GFP- and GFP-PARP13.2-overexpressing cells, suggesting that the Golgi defects were specific to PARP12 overexpression ( Supplementary Fig. S4B ). During mitosis, all CCCH Zn-finger PARPs localized to the cytoplasm ( Fig. 1c , Supplementary Fig. S2D ). Macro PARP9 and 14 were primarily cytoplasmic with additional nuclear localization consistent with previous studies ( Fig. 1b ) [28] , [29] , [30] . Nuclear PARP9 staining was highly enriched in S-phase-arrested cells ( Supplementary Fig. S1A,C ), suggesting that the previously described nucleocytoplasmic shuttling [28] of PARP9 might be cell cycle-regulated. In addition, PARP9 and 14 exhibited enriched localization at the cell periphery ( Fig. 1b ). Both proteins were later confirmed to co-localize with actin filaments, motile elements of the actin cytoskeleton that are enriched at the cell periphery ( Supplementary Fig. S3C ). Such enrichment was particularly prominent in cells fixed with 10% trichloroacetic acid (TCA), conditions ideal for staining cortical proteins [31] ( Supplementary Fig. S3C ). During mitosis, all macro PARPs were cytoplasmic; PARP9 staining was diffuse, whereas PARP14 staining was punctate ( Fig. 1c , Supplementary Fig. S2D ). Previous reports identified cytoplasmic localization for PARP4 (ref. 32 ), and cytoplasmic and nuclear localizations for PARP10, with a nuclear enrichment upon inhibition of nuclear export [33] . Each unclassified PARP localized to cytoplasm during interphase, with PARP4 and 11 exhibiting additional nuclear localization ( Fig. 1b ). PARP4 staining at the nucleus is likely non-specific as knockdown of PARP4 (see below) resulted in reduction of cytoplasmic, but not nuclear signal. PARP8 was enriched at the nuclear envelope in fixed cells ( Fig. 1b ), and cells expressing high concentrations of GFP-PARP8 exhibited nuclear accumulation of the protein ( Supplementary Fig. S1A,B ). PARP10 was punctate in the cytoplasm and largely absent from the nucleus. Similar to PARP13, PARP10 expression varied ∼ 6–7-fold among small clusters of cells ( Fig. 1b ). Cells with increased expression of PARP10 exhibited strong cytoplasmic juxtanuclear staining. Finally, PARP16 exhibited reticular membrane localization that co-localized with DiI, consistent with our previous results identifying it as an endoplasmic reticulum protein [7] ( Supplementary Fig. S3D ). Cells expressing high concentrations of GFP-PARP16 contained DiI-positive membrane structures as previously shown ( Supplementary Fig. S4C ) [7] . During mitosis, all unclassified PARPs localized throughout the cytoplasm. With the exception of PARP4, cytoplasmic staining was punctate ( Fig. 1c , Supplementary Fig. S2D ). PARP8 and 11 exhibited strong staining at the spindle poles as shown by co-staining with centrin ( Fig. 1c , Supplementary Fig. S3A ). No centriolar staining was identified for PARP11 during interphase, suggesting that the localization is specific to mitosis ( Fig. 1c , Supplementary Fig. S3A ). PAR is found throughout the cell The predominant cytoplasmic localization of the PARPs and their cell cycle-dependent localization patterns suggested that previously undetected cytoplasmic ADPr, generated in a cell cycle-dependent manner, could exist. Because reagents to label MAR are not well characterized [17] , [34] , we focused on PAR, for which several well-characterized antibodies are available. We examined PAR localization in asynchronous, G o /G 1 , S phase, and mitosis-arrested HeLa cells, and HeLa cells treated with H 2 O 2 to induce DNA damage, resulting in upregulated PAR synthesis in the nucleus [35] ( Fig. 2a , Supplementary Fig. S5A,C ). Cells were fixed with methanol (MeOH) or 20% TCA to minimize post-fixation PAR synthesis [36] and then stained with two antibodies generated against distinct PAR antigens: Tulip chicken anti-PAR IgY ( Fig. 2a ) and BD rabbit anti-PAR ( Supplementary Fig. S5C ). Cell cycle arrest was verified as above. Each fixation condition and antibody yielded similar results. Figure 2: Poly(ADP-ribose) is localized to the cytoplasm and nucleus throughout the cell cycle. ( a ) Asynchronous populations of HeLa cells (Asynch) or cells arrested in G 0 /G 1 , S phase or mitosis were fixed with MeOH or TCA and then stained for PAR (Tulip chIgY), and Centrin or γ-Tubulin, to identify single centriole pairs found during G o /G 1 , EdU, incorporated during S phase, and Tubulin, to stain mitotic spindles. In asynchronous cells and during G o /G 1 , S phase and mitosis, PAR staining was punctate with strong staining at the centrosome (arrowhead) and poles of the mitotic spindle (arrows). S-phase cells exhibited increased punctate staining in the nucleus relative to G o /G 1 cells. Merge shows PAR (red), cell cycle markers (green) and Hoechst 33342 (blue). Scale bars, 10 μm. ( b ) Cytoplasmic (C) and nuclear (N) extracts prepared from identical cell pellets, then normalized to cell volume, were generated from asynchronous, G o /G 1 and S-phase-arrested cells. Extracts were immunoblotted with Tulip chIgY anti-PAR antibody. Cytoplasmic and nuclear extracts were further examined for the presence of tubulin, a cytoplasmic protein, or PARP1, a nuclear protein, to assay for contamination between the fractions. Total cell extracts were also prepared from asynchronous (A) and mitotic (M) cells and immunoblotted with Tulip chIgY anti-PAR antibody. Positions of molecular-weight markers are indicated on the right in black, and molecular weights shown in italics identify the closest markers above and below the cropped region. ( c ) Quantitation of signal intensity of PAR immunoblots using chIgY and BD PAR antibodies. The ratio of nuclear to cytoplasmic PAR increases during S phase and DNA damage. The integrated intensity over the entire lane was determined, and the ratio of nuclear:cytoplasmic signal was calculated. Error bars represent s.d., n =3. See also Supplementary Fig. S5 . Full size image Significant amounts of PAR were detected in both cytoplasm and nucleus of asynchronous cells, H 2 O 2 -treated cells and during all cell cycle stages ( Fig. 2a , Supplementary Fig. S5A,C ). Staining in the interphase cytoplasm and nucleus appeared both diffuse and punctate, with increased nuclear PAR staining during S phase. Such staining was punctate and distinct from nuclear staining during other cell cycle stages, suggesting S-phase-specific functions for these puncta. In addition, PAR was also significantly enriched at the interphase centrosome and mitotic spindle poles, consistent with PARP localization described above and previous results [8] , [9] , [10] , [37] ( Fig. 2a , Supplementary Fig. S5C ). To biochemically validate cell cycle-dependent differences in PAR concentrations between the cellular compartments, the nuclear to cytoplasmic ratio of PAR was determined by generating nuclear and cytoplasmic extracts from H 2 O 2 -treated, asynchronous, and G o /G 1 - and S-phase-arrested cells. Extracts were immunoblotted with chIgY and BD anti-PAR ( Fig. 2b , Supplementary Fig. S5B,D ), and the nuclear to cytoplasmic PAR ratios were determined by integrating signal intensities of each lane of the blots ( Figs. 2c , n =3). During G o /G1, the ratio was 0.57±0.11 and 0.51±0.15 for the chIgY and BD PAR antibodies, respectively, and during S phase, this ratio increases to 1.3±0.33 and 1.2±0.39, respectively, for each antibody. During DNA damage, the ratio of nuclear to cytoplasmic PAR is 2.03±0.55 and 1.94±0.29 for chIgY and BD PAR antibodies, respectively. In addition, immunoblotting for PAR in asynchronous and mitotically arrested cells demonstrated increased PAR concentrations during mitosis, consistent with previous reports [10] ( Fig. 2b , Supplementary Fig. S5D ). Thus, significant amounts of PAR exist in the cytoplasm, and the relative amounts of PAR in the cytoplasm and nucleus change with the cell cycle. PARP-knockdown phenotypes We next examined the phenotypes of PARP knockdown via RNA interference (RNAi), focusing on changes in cell viability and morphology. For PARPs with unpublished phenotypes, at least eight small interfering RNAs (siRNAs) were generated. To verify phenotypes, at least two siRNAs demonstrating >80% protein knockdown via immunoblot and cell staining were required to result in similar phenotypes ( Figs. 3a,b , Supplementary Table S1 ). For PARPs 1, 2, 3, 4, 5a, 5b and 7, published siRNA sequences were utilized [9] , [38] . Published short hairpin RNA sequences for PARP10 knockdown [39] were ineffective in our siRNA assays; therefore, new siRNAs were screened. In all cases non-targeting siRNAs were used as control. 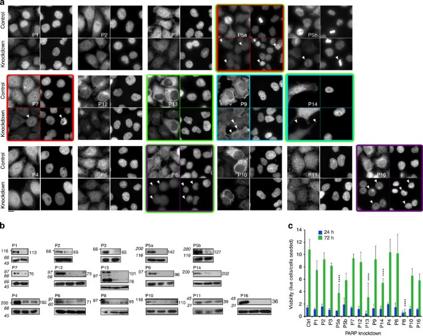Figure 3: Knockdown phenotypes of the PARP family. PARP-knockdown results in cell viability, membrane, actin cytoskeleton and mitosis phenotypes. PARP expression was knocked down via siRNA transfection in HeLa cells. Cells were then stained for each PARP (a) and immunoblot analysis performed to confirm knockdown (b). (a) Cells were transfected with control siRNAs (Control) or siRNAs specific for each PARP (knockdown) and then stained for PARP (left) and Hoechst 33342 (right). Knockdown identified four phenotypes: defects in membranes (purple boxes), actin cytoskeleton (cyan boxes), mitosis (red boxes) and cell viability (green boxes). Arrowheads indicate cells exhibiting knockdown. Scale bar, 10 μm. (b) Lysates from HeLa cells transfected with control (left lane) or PARP-specific siRNA (right lane(s)) were immunoblotted with corresponding anti-PARP antibody. Positions of molecular-weight markers are indicated on the right in black, molecular weights shown in italics identify the closest markers above and below the cropped region, and the approximate molecular weight (kDa) of the relevant PARP in each knockdown is indicated to the left of each PARP blot. The corresponding tubulin blot is included as a loading control (lower panels). (c) Cell number was analysed 24 and 72 h after knockdown of each PARP and presented as fold change relative to the initial number of cells seeded. PARP knockdowns that resulted in a decrease in viability of ≥2 s.d. relative to control knockdowns where identified as defective in cell viability. Error bars represent s.d.,n=3; ****P<0.00001, Student’st-test. See alsoSupplementary Fig. S6andTable 1. Figure 3: Knockdown phenotypes of the PARP family. PARP-knockdown results in cell viability, membrane, actin cytoskeleton and mitosis phenotypes. PARP expression was knocked down via siRNA transfection in HeLa cells. Cells were then stained for each PARP ( a ) and immunoblot analysis performed to confirm knockdown ( b ). ( a ) Cells were transfected with control siRNAs (Control) or siRNAs specific for each PARP (knockdown) and then stained for PARP (left) and Hoechst 33342 (right). Knockdown identified four phenotypes: defects in membranes (purple boxes), actin cytoskeleton (cyan boxes), mitosis (red boxes) and cell viability (green boxes). Arrowheads indicate cells exhibiting knockdown. Scale bar, 10 μm. ( b ) Lysates from HeLa cells transfected with control (left lane) or PARP-specific siRNA (right lane(s)) were immunoblotted with corresponding anti-PARP antibody. Positions of molecular-weight markers are indicated on the right in black, molecular weights shown in italics identify the closest markers above and below the cropped region, and the approximate molecular weight (kDa) of the relevant PARP in each knockdown is indicated to the left of each PARP blot. The corresponding tubulin blot is included as a loading control (lower panels). ( c ) Cell number was analysed 24 and 72 h after knockdown of each PARP and presented as fold change relative to the initial number of cells seeded. PARP knockdowns that resulted in a decrease in viability of ≥2 s.d. relative to control knockdowns where identified as defective in cell viability. Error bars represent s.d., n =3; **** P <0.00001, Student’s t -test. See also Supplementary Fig. S6 and Table 1. Full size image Cell viability was examined via seed assay in which PARPs were knocked down, total cell number was quantitated and cells were replated at the same density. Cell number was determined 24 or 72 h post seeding, and the ratio of cell number at each time point to initial seed number was used to assess defects in cell viability. PARP knockdowns that resulted in a fold change of at least two s.d. were considered to cause viability defects ( Fig. 3c ). Cell morphology was assayed by comparing PARP and DNA staining in control and knockdown cells and then verified by follow-up assays. In total, both assays identify four phenotypes upon PARP knockdown: decreased cell viability, defects in the actin cytoskeleton, defects in internal membrane structure and defects in mitosis. Knockdown of individual DNA-dependent PARPs did not result in observable changes in cell viability or morphological defects, suggesting that each is non-essential ( Figs. 3a,c ). PARP5a knockdown resulted in mitotic arrest, increased mitotic index confirmed by phosphoH3 staining ( ∼ 13% mitotic index in knockdown cells versus ∼ 3% in control) and decreased cell viability ( Fig. 3a,c ), consistent with our previous results and work by others [9] , [10] , [11] , [40] . PARP5b knockdown did not result in observable phenotypes or decreased viability ( Fig 3a,c ). Consistent with previous reports, PARP7 knockdown resulted in increased mitotic index confirmed by phosphoH3 staining ( ∼ 6% in knockdown cells versus ∼ 3% in control) [37] ( Fig. 3a , Supplementary Fig. S6 ). A significant decrease in cell viability was not observed in PARP7 knockdowns, suggesting that knockdown cells are able to undergo mitosis ( Fig. 3c ). Neither PARP12 nor 13 knockdown resulted in morphological phenotypes; however, PARP13 knockdown resulted in significantly decreased cell viability ( Fig. 3a,c ). Knockdown of each macro PARP resulted in cell morphology defects ( Fig. 3a ). Roughly, 25% of PARP9-knockdown cells exhibited pronounced membrane-blebbing phenotypes. This phenotype was not likely due to apoptosis, as a substantial increase in apoptotic nuclei, identified by the presence of highly condensed DNA via Hoescht staining, was not observed ( ∼ 3.5% in PARP9 knockdowns versus 1% in control) ( Fig. 3a ). PARP14 knockdown resulted in decreased cell viability ( Fig. 3c ) and dramatic alterations in cell morphology, as ∼ 60% of cells had elongated processes extending far from the cell body ( Fig. 3a , see below). Knockdown of PARP4, 6 and 10 did not result in obvious morphological defects or decreased cell viability ( Fig. 3a,c ). In contrast, PARP8 and 16 knockdown resulted in cell morphology defects, with ∼ 50% of PARP8- and ∼ 30% of PARP16-knockdown cells appearing completely round ( Fig. 3a ). PARP16-knockdown cells exhibiting the round cell phenotype were always found in pairs, whereas round PARP8 knockdowns were individual cells. PARP8 knockdown resulted in the most pronounced decrease in cell viability of all PARPs ( Fig. 3c ). PARP11 siRNAs were ineffective for knockdown, and therefore we cannot report on phenotype. PARP-knockdown phenotypes identify new cellular functions Cell morphology phenotypes identified in initial RNAi screens led us to design secondary assays to better understand function. Macro PARP knockdown phenotypes were reminiscent of actin cytoskeletal misregulation [41] , [42] . We therefore stained control, PARP9 and 14 knockdown cells with phalloidin, a filamentous actin (F-actin) label (PARP9 knockdowns), or an actin antibody (PARP14 knockdowns) ( Fig. 4 ). In control cells, PARP9 strongly co-localized with F-actin at the cell cortex, whereas PARP14 localized to the ends of actin fibres specifically at cell protrusions in a staining pattern consistent with FA structures ( Fig. 4 , arrowheads). Both PARP9 and 14 knockdowns exhibited highly abnormal F-actin staining, suggesting functions in actin cytoskeletal regulation; PARP9 knockdowns contained multiple actin-rich membrane blebs, and PARP14-knockdown cells exhibited highly elongated actin-rich processes ( Fig. 4 , arrows; Supplementary Fig. S3C ). These results are consistent with previous reports implicating this subfamily in the regulation of cell migration in B-cell lymphomas [43] . 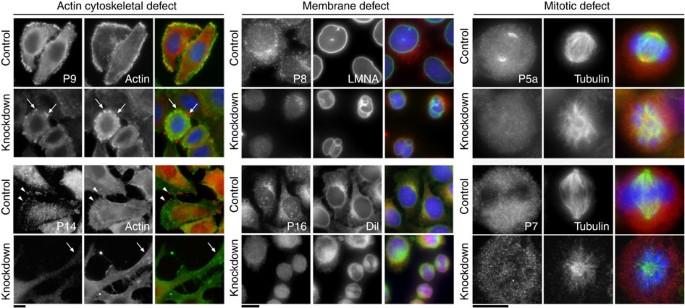Figure 4: Analysis of knockdown phenotypes identifies new PARP functions. Morphological phenotypes identified upon PARP knockdown were grouped into actin cytoskeletal, membrane or mitotic defects and then analysed to determine biological function. Control and knockdown cells stained with Hoechst 33342 (blue) and antibodies against the knocked down PARP (red). Cells exhibiting actin cytoskeletal defects were co-stained with phalloidin (P9) or an actin antibody (P14) to stain filamentous actin (green), membrane defects for lamin A/C (LMNA) or DiI (green) and mitotic defects for tubulin (green). PARP9 (P9) co-localized with actin in control cells. Knockdown resulted in actin-rich blebs shown by arrows. PARP14 (P14) localized to cell protrusions in control cells (arrowheads), identified inFig. 5as FAs. P14 knockdowns exhibited severe morphological defects with assembly of extended cellular protrusions (arrowheads). PARP8 (P8) co-localized with LMNA in control cells, but not knockdown cells. PARP8 knockdown resulted in abnormal, bilobed nuclei. PARP16 (P16) co-localized with the membrane dye DiI in control cells. Knockdown resulted in pairs of round cells. PARP5a (P5a), but not PARP7 (P7), localized to the mitotic spindle. Knockdown of P5a resulted in multipolar spindles, whereas P7 knockdown resulted in an increase in pre-metaphase spindles. Actin cytoskeletal defects are further examined inFigs. 5 and6, and mitotic defects inSupplementary Fig. S6. Scale bars, 10 μm. Figure 4: Analysis of knockdown phenotypes identifies new PARP functions. Morphological phenotypes identified upon PARP knockdown were grouped into actin cytoskeletal, membrane or mitotic defects and then analysed to determine biological function. Control and knockdown cells stained with Hoechst 33342 (blue) and antibodies against the knocked down PARP (red). Cells exhibiting actin cytoskeletal defects were co-stained with phalloidin (P9) or an actin antibody (P14) to stain filamentous actin (green), membrane defects for lamin A/C (LMNA) or DiI (green) and mitotic defects for tubulin (green). PARP9 (P9) co-localized with actin in control cells. Knockdown resulted in actin-rich blebs shown by arrows. PARP14 (P14) localized to cell protrusions in control cells (arrowheads), identified in Fig. 5 as FAs. P14 knockdowns exhibited severe morphological defects with assembly of extended cellular protrusions (arrowheads). PARP8 (P8) co-localized with LMNA in control cells, but not knockdown cells. PARP8 knockdown resulted in abnormal, bilobed nuclei. PARP16 (P16) co-localized with the membrane dye DiI in control cells. Knockdown resulted in pairs of round cells. PARP5a (P5a), but not PARP7 (P7), localized to the mitotic spindle. Knockdown of P5a resulted in multipolar spindles, whereas P7 knockdown resulted in an increase in pre-metaphase spindles. Actin cytoskeletal defects are further examined in Figs. 5 and6 , and mitotic defects in Supplementary Fig. S6 . Scale bars, 10 μm. Full size image The round cell phenotypes suggested that PARP8 and 16 knockdowns exhibited defects in membrane structure. Because of its nuclear envelope localization, we stained control and PARP8-knockdown cells with an antibody against the nuclear envelope protein Lamin A/C. PARP8 staining co-localized with Lamin A/C in control cells, and was largely undetectable at the nuclear envelope after PARP8 knockdown. The average size of nuclei in PARP8-knockdown cells was slightly smaller than control cells ( ∼ 180±50 μm 2 in knockdowns, n =360 cells versus 205±54 μm 2 in controls, n =282 cells). Lamin A/C staining identified multilobed nuclei in the knockdowns ( ∼ 14% in knockdowns versus 0.7% in controls, n >400 cells), suggesting structural defects in the nuclear envelope, or a misregulation of nuclear envelope biogenesis ( Fig. 4 ). Together, PARP8 localization to the nuclear envelope and the defects in nuclear envelope structure upon knockdown suggest that it is a critical nuclear envelope protein. PARP16 knockdown resulted in the accumulation of pairs of round cells, reminiscent of defective cytokinesis. PARP16 localization to membrane prompted us to examine membrane structure in the PARP16 knockdowns by staining with DiI ( Fig. 4 ). Total intensity of DiI staining was unchanged, however, PARP16 knockdowns exhibited a disruption of organized reticular membrane staining ( Fig. 4 ), perhaps a result of the dramatic change in cell morphology. It is unclear if this phenotype relates to PARP16 function in the unfolded protein response [7] ; however, activation of the unfolded protein response is known to result in cytokinesis defects in Saccharomyces cervisiae [44] . PARP5a and 7 knockdowns were stained for tubulin to examine spindle structure. Consistent with previous results, control cells exhibited PARP5a staining at spindle poles, and knockdown cells lacking PARP5a staining at spindle poles contained multiple microtubule foci and improperly aligned chromosomes ( ∼ 58% of mitotic cells with improperly aligned chromosomes for knockdowns versus 3% in controls, n >30 mitotic cells) [9] , [10] , [40] ( Fig. 4 , Supplementary Fig. S6 ). In contrast, PARP7 did not localize to the mitotic spindle in control cells. Tubulin staining of PARP7 knockdowns revealed a disproportionate increase in pre-metaphase cells among mitotic cells ( ∼ 57% in PARP7 knockdown versus ∼ 19% in controls, n >50 mitotic cells), a mitotic defect distinct from that of PARP5a knockdown ( Fig. 4 , Supplementary Fig. S6 ). As the increase in mitotic index was mild ( ∼ 6% versus ∼ 3% for control cells) and PARP7 knockdown did not significantly decrease cell viability, our results suggest that PARP7 is not required for spindle function, but that its knockdown increases the length of pre-metaphase mitosis. PARP14 is a focal adhesion protein The PARP14 knockdown phenotype was particularly striking, prompting us to closely examine its function in actin cytoskeletal regulation. Both PARP14 siRNAs resulted in cells that were elongated and contained dendritic-like membrane protrusions emanating from the cell body ( Figs. 5a,b ). These extended cellular protrusions were substantial PARP14 knockdowns measured ∼ 3 times longer than control cells ( n =20 cells) ( Fig. 5b ). Greater than 60% of PARP14 knockdown cells exhibited these extended protrusions in contrast to control knockdown cells that contained similar protrusions in ∼ 5% of the population ( n =3, 200 cells counted for each condition) ( Fig. 5b ). 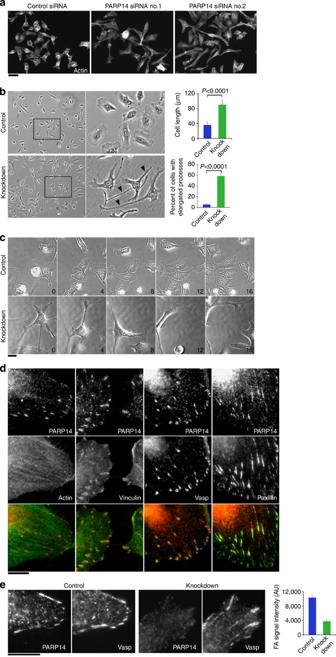Figure 5: PARP14 is a FA protein whose knockdown results in abnormal cell morphology and cell migration defects. (a) HeLa cells were transfected with control siRNA or siRNA 1 or 2 directed against distinct PARP14 sequences and then stained with phalloidin. Both PARP14 siRNAs result in similar cell phenotypes containing extended cellular protrusions. Scale bar, 50 μm. (b) Bright field images of representative fields of control and PARP14 siRNA-treated cells. Extended cellular protrusions in PARP14 siRNA-treated cells are marked with arrowheads. Quantitation of maximum cell length (n=20 cells) and percentage of cells displaying extended cellular protrusions (n=3, 200 cells counted per condition) are shown at left. Error bars represent s.d. Significance determined by Student’st-test. (c) Still images of the indicated time points of movies taken of control and PARP14 siRNA-treated cells undergoing random migration on the substrate fibronectin. See alsoSupplementary Movie 1(control cells) andSupplementary Movie 2(PARP14-depleted cells). Scale bar, 25 μm. (d) HeLa cells were plated on fibronectin fixed with TCA and stained for PARP14 (red) and the indicated FA proteins (green). Scale bar, 10 μm. (e) Control and PARP14-knockdown cells were fixed with TCA and co-stained for PARP14 and VASP. PARP14 knockdown results in loss of signal at FAs demonstrating the specificity of FA staining (arrows). The intensity of PARP14 signal at FAs was quantified in both control and PARP14-knockdown cells. Scale bar, 10 μm. Figure 5: PARP14 is a FA protein whose knockdown results in abnormal cell morphology and cell migration defects. ( a ) HeLa cells were transfected with control siRNA or siRNA 1 or 2 directed against distinct PARP14 sequences and then stained with phalloidin. Both PARP14 siRNAs result in similar cell phenotypes containing extended cellular protrusions. Scale bar, 50 μm. ( b ) Bright field images of representative fields of control and PARP14 siRNA-treated cells. Extended cellular protrusions in PARP14 siRNA-treated cells are marked with arrowheads. Quantitation of maximum cell length ( n =20 cells) and percentage of cells displaying extended cellular protrusions ( n =3, 200 cells counted per condition) are shown at left. Error bars represent s.d. Significance determined by Student’s t -test. ( c ) Still images of the indicated time points of movies taken of control and PARP14 siRNA-treated cells undergoing random migration on the substrate fibronectin. See also Supplementary Movie 1 (control cells) and Supplementary Movie 2 (PARP14-depleted cells). Scale bar, 25 μm. ( d ) HeLa cells were plated on fibronectin fixed with TCA and stained for PARP14 (red) and the indicated FA proteins (green). Scale bar, 10 μm. ( e ) Control and PARP14-knockdown cells were fixed with TCA and co-stained for PARP14 and VASP. PARP14 knockdown results in loss of signal at FAs demonstrating the specificity of FA staining (arrows). The intensity of PARP14 signal at FAs was quantified in both control and PARP14-knockdown cells. Scale bar, 10 μm. Full size image To better understand how these extended protrusions were generated, we analysed control and PARP14 knockdowns using real-time imaging. In control cells, small membrane protrusions were generated and quickly retracted as cells moved in different directions ( Fig. 5c , Supplementary Movie 1 ). In PARP14 knockdowns, cells appeared unable to retract protrusions efficiently, resulting in highly elongated extensions ( Fig. 5c , Supplementary Movie 2 ). Thus, abnormal membrane protrusions appeared to result from defective retraction of protrusions normally generated in migrating cells. Retraction of protrusions was so defective in PARP14 knockdowns that cells stretched into severely elongated shapes as they explored the substrate ( Fig. 5c , Supplementary Movie 2 ). A major control point in cell migration is the assembly, maturation and disassembly of FAs, multi-protein complexes that serve as connections between the substrate and the actin cytoskeleton [45] . FA regulation requires the ordered recruitment of FA proteins, and the strength and stability of FAs depend on the protein composition of the FA [46] . Cells must balance FA strength so that adhesions are strong enough to pull the cell forward, but sufficiently labile so that they can be rapidly disassembled as the cell moves. The PARP14-knockdown phenotype suggested defects in FA function. A previous proteomic study identified PARP14 protein in purified FAs isolated from HFF-1 cells [46] , consistent with the PARP14 staining at cell protrusions we observed ( Fig. 4 , Supplementary Fig. S3C ). We therefore examined PARP14 localization at FAs in HeLa cells grown on fibronectin-coated coverslips (to mimic extracellular substrate). Cells were fixed and stained with antibodies against PARP14 and known FA components. PARP14 localized to the ends of actin stress fibres, similar to other FA proteins, and co-localized with vinculin, vasodilator-stimulated phosphoprotein (VASP) and paxillin ( Fig. 5d ). The specificity of PARP14 localization at FAs was confirmed by examining PARP14 antibody staining at FAs after targeted knockdown ( Fig. 5e ). PARP14 knockdown resulted in near-complete depletion of PARP14 staining at FAs, whereas VASP staining was maintained. In addition to validating the specificity of PARP14 localization to the FA, this result also indicates that PARP14 is not required for general FA assembly ( Fig. 5e . Importantly, such siRNA treatments did not deplete cytoplasmic or nuclear PARP14 staining, suggesting that staining at these locations is either non-specific or represents siRNA-resistant populations of PARP14. PARP14 regulates focal adhesion function For cells to properly retract membrane protrusions, they must be able to efficiently breakdown FAs in a process called FA turnover [47] . The inability of PARP14-knockdown cells to properly retract membrane protrusions, combined with its localization to FAs, suggested that PARP14 functions in FA turnover. Therefore, we examined FA adhesive force in control and PARP14 knockdowns using three independent assays. First, we utilized a trypsin-based detachment assay measuring time required to detach cells from substrate [48] . PARP14-knockdown cells were more resistant to trypsinization than controls, with ∼ 2 times more cells remaining adhered after similar periods of trypsinization ( Fig. 6a ). Second, we employed a centrifugation assay comparing the number of cells remaining adhered to substrate after constant application of centrifugal force. Approximately five times more PARP14-knockdown cells remained adhered to substrate after centrifugation compared with controls ( Fig. 6b ). Third, we used a cell-spreading assay measuring the area of cell spreading per unit time ( Fig. 6c ). At early time points when cells adhered to substrate but had not yet formed defined FAs, control and PARP14 knockdowns were of similar size, suggesting that the morphological defects observed in PARP14 knockdowns were dependent on FA formation and not simply a property of the cells themselves. As cells assembled FAs and spread onto substrate, PARP14-knockdown cells covered ∼ twice the surface area of control cells at each time point ( Fig. 6c ). These three independent assays suggest that the adhesive strength between FAs and substrate is stronger in PARP14 knockdowns relative to control. It is likely that this increased adhesive strength leads to slowed FA disassembly and prevents cellular protrusions from properly retracting. 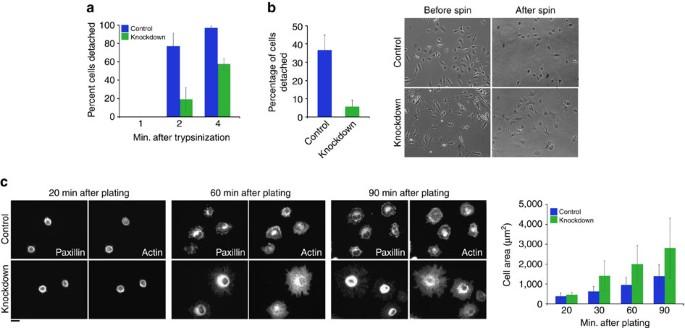Figure 6: PARP14 depletion from FAs results in increased adhesive strength. (a) Control or PARP14 siRNA-treated cells plated on fibronectin were treated with trypsin for the indicated times, and percentage of cells detached was quantified at each time point. Error bars represent s.d. (b) Control or PARP14 siRNA-treated cells plated on fibronectin were subjected to a constant centrifugal force (2,000g) for 30 min, and the number of cells detached during centrifugation was quantified. Representative images of control and PARP14-knockdown cells before and after centrifugation shown at right. Error bars represent s.d. (c) Control or PARP14 siRNA-treated cells were allowed to adhere to a fibronectin-coated plate for the indicated times, fixed and stained with anti-paxillin and phalloidin, and the area of individual cells was quantified at each time point. Error bars represent s.d. Representative images of control or PARP14-knockdown cells at each time point are shown. Scale bar, 25 μm. Figure 6: PARP14 depletion from FAs results in increased adhesive strength. ( a ) Control or PARP14 siRNA-treated cells plated on fibronectin were treated with trypsin for the indicated times, and percentage of cells detached was quantified at each time point. Error bars represent s.d. ( b ) Control or PARP14 siRNA-treated cells plated on fibronectin were subjected to a constant centrifugal force (2,000 g ) for 30 min, and the number of cells detached during centrifugation was quantified. Representative images of control and PARP14-knockdown cells before and after centrifugation shown at right. Error bars represent s.d. ( c ) Control or PARP14 siRNA-treated cells were allowed to adhere to a fibronectin-coated plate for the indicated times, fixed and stained with anti-paxillin and phalloidin, and the area of individual cells was quantified at each time point. Error bars represent s.d. Representative images of control or PARP14-knockdown cells at each time point are shown. Scale bar, 25 μm. Full size image The initial bioinformatic identification of 17 human PARP genes suggested that PARPs function in more biological pathways than previously imagined [14] , [49] . Our analysis confirms the diversity of PARP function and leads to several important conclusions regarding the protein family. First, nearly all (16 out of 17) of the PARPs predicted to exist in humans are expressed in epithelial cells collected from the retina and cervical tumours tissues of diverse origin. This suggests ubiquitous expression of most PARPs among human tissues. Second, PARPs are predominantly cytoplasmic proteins, and a significant amount of one product of PARP activity, PAR, is present in the cytoplasm. Third, PAR synthesis/hydrolysis appears to be cell cycle-regulated as the ratio of PAR synthesis/hydrolysis in the nucleus and cytoplasm changes during specific cell cycle stages. This suggests cell cycle-specific functions for PAR. Finally, PARP proteins are important regulators of somatic cell physiology and function in multiple diverse pathways. The importance of nuclear PARP function in the physiology of the cell is well established. PARP1/PARP2 regulate critical physiological functions in the nucleus, and although neither PARP1 nor PARP2 are essential for life [50] , PARP1/2 double-knockout mice are non-viable, suggesting that the activity of a least one of these PARPs is essential [51] . Our data suggests that PARP function in the cytoplasm is equally important. All multicellular eukaryotes encode both nuclear and cytoplasmic PARPs with vertebrates containing the most PARPs [52] . The additional PARPs found in vertebrates are cytoplasmic, and each PARP identified as essential for cell viability is found in the cytoplasm of all vertebrates, suggesting that vertebrate evolution led to an increased requirement for cytoplasmic PARP function [52] . Each of the PARP-knockdown phenotypes points to a remarkable diversity of function among this family of proteins. Such diversity is likely conferred by the diverse functional domains present outside of the conserved PARP domain, such as the DNA-binding domains of DNA-dependent PARPs, and the ADPr-binding macro domains of the macro PARPs [17] . The similarity of localization and function of subfamily members demonstrate the importance of these functional domains and suggest that in addition to previously described roles in regulation of PARP enzymatic activity [53] , [54] , they can target PARPs to specific cellular locations ( Fig. 1a and Table 1 ). The defects in cell viability in PARP5a, 8 and 14 knockdowns are not surprising, given their phenotypes. In contrast, PARP13 knockdowns did not result in obvious morphological defects, thus its requirement for cell viability is unclear. PARP13 has been shown to be an important regulator of mRNA, targeting viral RNA for degradation and regulating cellular mRNA post-transcriptionally by regulating miRNA activity [6] , [55] . Because cell cycle progression is regulated by miRNA activity [56] , it is possible that the decreased cell viability resulting from PARP13 knockdown results from misregulation of miRNA function or that the cell viability defect is due to general misregulation of mRNA metabolism. Our PARP8, 12 and 16 data suggest potential functions for PARPs in the assembly or maintenance of membranous organelles. Each of the structures to which PARP8, 12 and 16 localize are derived from endoplasmic reticulum, and requires trafficking from the endoplasmic reticulum for function, processes regulated by glycosylation [57] . Perhaps ADPr could serve a similar function as glycosylation in vesicle trafficking either by functioning as a trafficking signal or by regulating glycosylation of target proteins. Finally, macro PARPs had been postulated to regulate B-cell motility via unknown mechanisms, with overexpression of PARP9 resulting in increased migration of B-cell lymphomas [43] . Our results provide a potential explanation for these observations by demonstrating that macro PARPs localize to the motile elements of the actin cytoskeleton and exhibit cytoskeletal defects upon knockdown. Interestingly, PARP14 expression is upregulated in multiple myelomas and has been shown to regulate the expression of IL-4 and B-cell survival factors [58] , [59] . As such, PARP14 has been mentioned as a possible target for therapeutic inhibition of multiple myelomas. It is unclear if there is a connection between this specific PARP14 function in these specialized cell types and PARP14 function at FAs. However, it is possible that inhibiting the enzymatic activity of PARP14 could also affect cellular adhesiveness, making PARP14 an attractive target for the therapeutic inhibition of metastatic cancers in addition to multiple myelomas. Cell culture and reagents Cells were grown at 37 °C and 5% CO 2 . HeLa cells (ATCC) were passaged in DMEM+10% FBS (Tissue Culture Biologicals)+penicillin/streptomycin (Invitrogen); hTERT-RPE1 cells (ATCC) in Ham’s F12/DMEM (1:1) (Mediatech)+10% FBS, penicillin/streptomycin and 0.01 mg ml −1 hygromycin B (Invitrogen). Anti-PARP peptide antibodies were generated and affinity-purified using a standard protocol [60] . Antibodies (stored at 1 mg ml −1 ) were used at 1:100 for immunofluorescence (IF) and 1:1,000 for immunoblot (IB). Additional antibodies used were anti-pADPr (chIgY, Tulip Biolabs, 1:100 IF, 1:500 IB; 51–811KD, BD Pharmingen, 1:100 IF, 1:500 IB), anti-PARP1 (PA3-951, Affinity Bioreagents, 1:1,000 IB), anti-PARP5a (H350, Santa Cruz Biotechnology, 1:100 IF, 1:1,000 IB), anti-PARP14 (HPA012063, 1:100 IB; HPA008846, 1:100 IF, Sigma-Aldrich), anti-GFP (ab1218, Abcam, 1:100 IF; JL8, Clontech, 1:2,500 IB), anti-Tubulin (YL1/2, Abcam, 1:1,000 IF, 1:5,000 IB), anti-lamin A/C (ab8984, Abcam, 1:100 IF), anti-actin (A3853, Sigma-Aldrich, 1:100 IF), anti-vasp (a kind gift from F. Gertler, 1:500 IF), anti-zyxin (ab71842, Abcam, 1:200 IF), anti-paxillin (610051, BD Biosciences, 1:1,000 IF), anti-vinculin (Sigma-Aldrich, 1:200 IF), anti-p230 (611280, BD Transduction Laboratories, 1:200), anti-gamma tubulin (GTU88, Sigma-Aldrich, 1:10,000 IF), anti pH2AX (05-636, Millipore, 1:100 IF), anti-centrin (a kind gift from J. Salisbury, 1:1,000 IF) and anti-SBP (ab119491, Abcam, 1:500 IF). Secondary antibodies, phalloidin, DiI, EdU labelling kit and Hoechst 33342 were from Invitrogen. siRNA oligonucleotides were purchased from Invitrogen (Stealth or Silencer Select) or Dharmacon (siGenome) ( Table S1 ). Transfections HeLa cells were transfected using Lipofectamine 2000 (Invitrogen) according to the manufacturer’s protocols. For RNAi of PARPs 1–4, HeLa cells were transfected with 20 nM siRNA for at least 24 h before splitting onto coverslips. Knockdown analysis was performed 48 h post transfection. For PARPs 5a–16, HeLa cells were transfected with 20 nM siRNA for at least 24 h. Cells were split and re-transfected the following day with identical concentrations of siRNA for 24 h before splitting. Knockdown analysis was performed 96 h after initial transfection. AllStars negative control siRNA (Qiagen) was used as control. For further validation of PARP14-knockdown phenotype, HeLa cells were transfected with 25 nM siRNA and allowed to incubate in transfection mixture for at least 48 h before splitting. Immunofluorescence For all transfections, cells were plated on coverslips 6 h post transfections. For G 0 /G 1 arrests, cells were plated at 50% confluence and serum starved for 72 h. For S-phase arrest, cells were treated with 5 μg ml −1 aphidicolin for 16 h. For mitotic arrest, cells were treated with either 200 or 400 nM nocodazole for 16 h. Coverslips were fixed in either −20° MeOH for 5 min, 10 or 20% TCA (Fluka) for 15 min at 4°, or 4% formaldehyde (Polysciences) in PBS (Invitrogen) for 15 min followed by extraction with 0.5% Triton X-100 (Sigma) in PBS for 10 min. For validation of PARP14 localization, cells were grown on fibronectin-coated coverslips and fixed in 10% TCA. Coverslips were blocked in abdil (PBS containing 4% BSA, 0.1% Triton X-100 and 0.02% sodium azide) and then incubated with primary and secondary antibodies for 45 min. All antibody dilutions were generated in abdil. For quantitation of Golgi area in PARP12 overexpression and nuclear area in PARP8 knockdowns, NIS-Elements software was used to generate a region of interest around the Golgi/nucleus, and the area of the region of interest was determined. Viability assay Following RNAi knockdown, cells were counted using a Cellometer automated cell counter and then normalized and split in duplicate. Living cells were then counted after 24 and 72 h using trypan blue exclusion and a Cellometer automated cell counter. Viability was assessed by calculating the fold change in cell number relative to cell number initially seeded. PARPs whose knockdown resulted in a decrease in fold change compared with control knockdown of at least two s.d. were considered to have an effect on viability. Three independent experiments were performed for viability analysis. Real-time imaging Control and PARP14-knockdown HeLa cells were split into six-well glass bottom plates (Greiner Bio-One) coated with fibronectin and grown overnight. Cells were rinsed with PBS and changed into CO 2 -independent medium containing 10% FBS (Invitrogen) for imaging. Bright field images were collected every 5 min for 16 h. All live imaging was performed using a Nikon TiEclipse microscope equipped with an environmental chamber with CO 2 and temperature control and Hamamatsu ORCA R 2 digital camera. Cell adhesion assays For trypsin-based assays, cells were sparsely seeded onto fibronectin-coated plates and then incubated overnight. The next morning, the number of cells in each well was calculated. Cells were washed 2 × with PBS and then treated with 0.025% trypsin in DMEM. At the indicated time points, the number of cells released into the media and the number of cells remaining on the plate were counted. For centrifugal-based assays, cells were sparsely seeded onto fibronectin-coated plates and then incubated overnight. The next morning, the number of cells in each well was calculated. Cells were washed 3 × with PBS and then centrifuged inverted for 30 min at 2,000 g . The number of cells remaining in each well after centrifugation was then counted. For cell-spreading assays, plated cells were gently trypsinized, resuspended in DMEM and then allowed to recover for 10 min at 37 °C. Cells were then very sparsely seeded onto fibronectin-coated coverslips. At the indicated time points after plating, coverslips were gently washed with PBS, then fixed and stained. RNA sequencing Total RNA was purified from HeLa and hTERT-RPE1 cells using a Qiagen RNeasy kit. The samples were poly-A-purified, and cDNA libraries were synthesized using the Illumina Tru-Seq protocol. The libraries were sequenced on Illumina HiSeq2000 obtaining 40-nt single-end reads. The reads were mapped to the Human genome (hg19) using bowtie2 version 2.0.0-beta6, samtools version 0.1.18 and tophat version 2.0.4. How to cite this article: Vyas, S. et al. A systematic analysis of the PARP protein family identifies new functions critical for cell physiology. Nat. Commun. 4:2240 doi: 10.1038/ncomms3240 (2013)